Opposing effects of target overexpression reveal drug mechanisms Overexpression of a drug’s molecular target often increases drug resistance, offering a pathway for adaptive evolution and a tool for target identification. It is unclear though why this phenomenon applies to some drugs but not others. Here we gradually overexpressed antibiotic targets in Escherichia coli and found that drug resistance can increase, remain unchanged, decrease or even change non-monotonically. Even a single target can produce opposing responses to its different inhibitors. We explain these contradicting effects with quantitative models of enzyme inhibition that account for fitness costs and the biochemical activity or inactivity of drug–enzyme complexes. Thus, target overexpression confers resistance or sensitivity as a predictable property of drug mechanism, explaining its variable presence in nature as a resistance mechanism. Though overexpression screens may fail at identifying unknown targets, overexpressing known or putative targets provides a systematic approach to distinguish between simple inhibition and complex mechanisms of drug action. Resistance to growth-inhibitory drugs can often be conferred by overexpression of the gene encoding a drug’s molecular target. When this is true, two important results follow. First, in bacteria, protozoa, plants, insects and tumour cells alike, drug resistance can evolve by gene amplification or overexpression of the drug’s target [1] , [2] , [3] , [4] , [5] , [6] , [7] , [8] . Second, unknown drug targets can be identified by screening for drug resistance among overexpression mutants [9] , [10] , [11] , [12] , [13] , [14] , [15] , [16] . A variety of experimental methods for drug target identification are founded on the hypothesis that target overexpression confers drug resistance, or that target knockdown (that is, underexpression) should confer drug susceptibility. The rationale is simple: when more or fewer copies of the target are present, a higher or lower drug concentration is required to reduce the total target activity below the level required for cell viability or growth [14] , [15] , [16] , [17] , [18] , [19] . These hypotheses, however, do not appear to hold true for all drugs: for many drugs clinical resistance is never reported as a result of target gene amplification [4] , [19] , [20] , [21] , and small molecule target identification remains a major challenge in pharmaceutical development. Despite the evolutionary and pharmacological importance of resistance by target overexpression, it remains unclear why this phenomenon is only seen for some drugs but not others. Here we address this question by examining antibiotics with known targets in Escherichia coli . For some drugs, resistance cannot result from ‘target gene’ overexpression because no such single gene exists. A drug’s efficacy can depend on binding multiple targets (for example, many beta-lactams and kinase inhibitors), or a drug can act on non-protein targets (for example, polymyxins, vancomycin, DNA intercalators). The question of overexpression-mediated resistance is therefore most relevant and well defined for drugs with a single protein target. 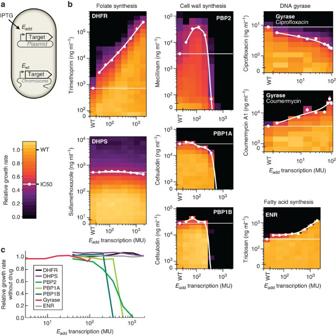Figure 1: Overexpression of a drug’s target gene can increase, decrease or have no effect on drug resistance. (a)E. colistrains were constructed with IPTG adjustable overexpression of drug target genes. (b) For each drug–gene pair, bacterial growth rates (heatmap) were measured over gradients of drug dose (vertical axis) and IPTG-induced gene dose (horizontal axis). Transcript overexpression (Eadd) was quantified in Miller Units (MU) from kinetic beta-galactosidase assays of a strain whose plasmid encodedlacZinstead of a drug target, grown in the absence of drug. At eachEaddlevel, the IC50 (drug concentration that inhibits growth to 50% of uninhibited wildtype growth) is shown (white dots and trend line) and compared with the IC50 of the wildtype (thin flat white line; WT denotes strain with empty plasmid). (c) Drug target genes incur variable fitness costs when overexpressed, even in the absence of drugs. We identified six such antibiotics with a single protein-based target and also included a beta-lactam, cefsulodin, selective for two paralogs of the penicillin-binding protein, PBP1 [22] ( Table 1 ). Table 1 List of drugs and drug targets utilized in this study. Full size table We find that overexpressing antibiotic targets in bacteria can cause both positive and negative changes in drug resistance, and we use mathematical models to show that these effects depend on whether a drug merely inhibits its target or induces harmful target-catalyzed reactions. Thus gene overexpression can fail at identifying what is a drug’s target, but overexpressing known targets provides a systematic method to reveal how a drug affects its target. Target overexpression has conflicting effects on drug resistance For each target–drug pair, we measured the level of resistance as a function of increasing target overexpression. We constructed strains that overexpress the target genes from an isopropyl β- D -1-thiogalactopyranoside (IPTG)-inducible promoter and calibrated transcription rate by beta-galactosidase assays ( Fig. 1a and Supplementary Fig. 1 ) [25] , [26] . Beta-galactosidase assays under partially inhibitory doses of each of the antibiotics in this study revealed that the IPTG-induction system is robust to these perturbations ( Supplementary Fig. 2 ). DNA Gyrase was overexpressed from a transcript encoding both subunits ( gyrA and gyrB ). At each of several target overexpression levels, we measured bacterial growth rates over a range of drug concentrations using a sensitive bioluminescence-based assay [27] to quantify how drug resistance is altered. Figure 1: Overexpression of a drug’s target gene can increase, decrease or have no effect on drug resistance. ( a ) E. coli strains were constructed with IPTG adjustable overexpression of drug target genes. ( b ) For each drug–gene pair, bacterial growth rates (heatmap) were measured over gradients of drug dose (vertical axis) and IPTG-induced gene dose (horizontal axis). Transcript overexpression ( E add ) was quantified in Miller Units (MU) from kinetic beta-galactosidase assays of a strain whose plasmid encoded lacZ instead of a drug target, grown in the absence of drug. At each E add level, the IC50 (drug concentration that inhibits growth to 50% of uninhibited wildtype growth) is shown (white dots and trend line) and compared with the IC50 of the wildtype (thin flat white line; WT denotes strain with empty plasmid). ( c ) Drug target genes incur variable fitness costs when overexpressed, even in the absence of drugs. Full size image Overexpression of target genes had qualitatively different effects on drug resistance ( Fig. 1b ). The drug concentration that inhibits growth by 50% (IC50) was increased by expressing the targets of trimethoprim (Dihydrofolate reductase (DHFR)), triclosan (enoyl-acyl carrier protein reductase (ENR)), and coumermycin A1 (Gyrase) but decreased when expressing the targets of ciprofloxacin (Gyrase) and cefsulodin (penicillin binding protein 1A (PBP1A) and PBP1B; though low PBP1B expression conferred a minor increase in IC50). Resistance to sulfamethoxazole, a sulphonamide antibiotic, was independent of target (Dihydropteroate synthase (DHPS)) expression level, and the IC50 of mecillinam increased substantially with mild target (PBP2) overexpression but decreased with stronger overexpression. The presence or absence of resistance from target overexpression is consistent with clinically-observed mechanisms of resistance. Bacteria resistant to trimethoprim or triclosan have been reported with elevated target expression or promoter mutations in the target [2] , [5] . Conversely, though many mutants resistant to sulphonamides or ciprofloxacin have been characterized, no resistance-conferring amplifications or ‘promoter-up’ mutations in the targets have been reported [20] , [21] . A model of drug resistance due to target overexpression We sought to understand the relation between drug resistance and drug target expression levels using simple mathematical models of enzyme overexpression which account for the mechanisms of drug action and the fitness costs of gene expression. First, considering enzyme inhibition, we built mass-action models of competitive and non-competitive inhibition and calculated how drug susceptibility is affected by enzyme overexpression. We assume that 50% growth inhibition (IC50) occurs when the flux through an essential enzyme is inhibited by factor of 2. In reality this relationship varies between drug targets [28] , but any other value yields similar results in our model ( Supplementary Fig. 3 ; also, a drug-induced change in substrate concentration yields similar results). These models yield a linear dependence of IC50 on the fold overexpression of the enzyme ( Fig. 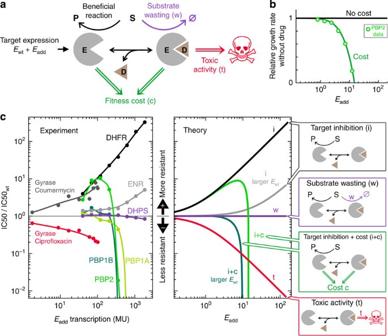Figure 2: Drug mechanism of action and fitness costs of target overexpression define the diverse changes in resistance when drug targets are overexpressed. (a) Mass-action models of enzyme inhibition quantified the relation between drug concentration, growth inhibition and enzyme expression (wildtype expression=Ewt, additional expression=Eadd; arbitrary units). Model variants explored different mechanisms of drug action: inhibition of a beneficial reaction, wasting of an essential substrate, and enzyme–drug complexes that actively exert a toxic effect. Also modelled was the effect of some drug targets to incur fitness costs when overexpressed. (b) The following models use a cost function (green line) based on the experimentally observed costs of PBP2 overexpression (circles; 1 model unit ofEadd=50 MU). (c) Simple models that consider different mechanisms of drug action produce diverse changes in resistance as drug targets are overexpressed, thus rationalizing the conflicting experimental observations, the variable presence in nature of drug resistance by target overexpression, and presenting a tool to investigate drug mechanism of action. 2 , model i; Supplementary Methods ): Figure 2: Drug mechanism of action and fitness costs of target overexpression define the diverse changes in resistance when drug targets are overexpressed. ( a ) Mass-action models of enzyme inhibition quantified the relation between drug concentration, growth inhibition and enzyme expression (wildtype expression= E wt , additional expression= E add ; arbitrary units). Model variants explored different mechanisms of drug action: inhibition of a beneficial reaction, wasting of an essential substrate, and enzyme–drug complexes that actively exert a toxic effect. Also modelled was the effect of some drug targets to incur fitness costs when overexpressed. ( b ) The following models use a cost function (green line) based on the experimentally observed costs of PBP2 overexpression (circles; 1 model unit of E add =50 MU). ( c ) Simple models that consider different mechanisms of drug action produce diverse changes in resistance as drug targets are overexpressed, thus rationalizing the conflicting experimental observations, the variable presence in nature of drug resistance by target overexpression, and presenting a tool to investigate drug mechanism of action. Full size image where E wt is the wildtype enzyme abundance and E add is the additional (overexpressed) quantity of enzyme. Simply put, if the enzyme is overexpressed 10-fold then 50% flux inhibition requires 95% enzyme inhibition. Second, we accounted for the strong fitness costs that the overexpression of some drug targets incur even in the absence of drug ( Figs 1c and 2b ). The fitness costs of gene expression are gene and context dependent, and can arise from many sources including the process and energetic costs of gene expression and localization, the presence or activity of specific proteins, and from the consequences of misfolding or aggregation [29] , [30] , [31] , [32] . Regardless of their specific origin, if severe fitness costs are incurred by the overexpression of a drug’s target, they can present an obstacle to the acquisition of drug resistance by target overexpression. Including a fitness cost as an additive mechanism of toxicity [33] yields ( Fig. 2 , model i+c; Supplementary Methods ): This inhibition-cost model applies most readily to drugs that simply inhibit their target, and indeed it describes the observed changes in resistance for the antibiotics of such a mechanism [22] , [34] , [35] , [36] , [37] , [38] . Specifically, it rationalizes both the monotonic increase in resistance observed for the drug–target pairs trimethoprim–DHFR, triclosan–ENR and coumermycin A1–Gyrase (Fig. 2 , model i), as well as the non-monotonic response displayed by mecillinam–PBP2 ( Fig. 2 , model i+c). For cefsulodin, its inhibition of two targets, PBP1A and PBP1B, must be considered: neither target is an essential gene, but the inhibition or deletion of both is lethal [22] , [39] . Biochemical and genetic studies show that growth at the brink of cefsulodin inhibition depends on PBP1B function: PBP1A binds to cefsulodin with 10-fold higher affinity than does PBP1B, and PBP1B deletion dramatically heightens the sensitivity of E. coli to cefsulodin whereas PBP1A deletion has no effect [39] , [40] , [41] . These properties indicate that the current model should apply to PBP1B – the growth-limiting target of cefsulodin – consistent with the observation that PBP1B but not PBP1A overexpression is able to confer any cefsulodin resistance before lethal fitness costs are incurred by overexpression ( Fig. 1b ). This model also shows that because resistance depends on the relative magnitudes of E add and E wt , differences in E wt between targets can explain the quantitative difference in IC50 changes between trimethoprim–DHFR and triclosan–ENR ( Supplementary Fig. 4 ). In summary, for enzyme-inhibiting drugs, target overexpression can confer resistance by compensating for inhibition, but the potential for resistance may be limited if overexpression is costly. Why are some drugs never resisted by target overexpression? A target gene might be very costly to express at any amount greater than wildtype, permitting no opportunity for protective overexpression. A protein may fail to fold at higher expression levels than wildtype, in which case both artificial expression systems and naturally occurring overexpression mutants may fail to produce more functional target. However, these scenarios do not explain why sulfamethoxazole resistance is unchanged by non-costly DHPS overexpression (which can be overexpressed in E. coli to 7000-fold greater specific activity [42] ), nor why ciprofloxacin resistance decreases with non-costly Gyrase overexpression. These cases are particularly intriguing given that other drugs affecting the same gene or pathway are resisted by target overexpression. Trimethoprim, like sulfamethoxazole, inhibits folate synthesis, but is resisted by target overexpression (DHFR). Coumermycin A1, like ciprofloxacin, binds to Gyrase, but is resisted by Gyrase overexpression. To understand how seemingly subtle differences between molecular mechanisms of drug action can define whether or not target overexpression confers resistance, we next explain these contrasting behaviours. Target overexpression does not resist drugs that divert flux The qualitatively different responses of trimethoprim and sulfamethoxazole to target overexpression arise from a specific difference between their chemical mechanisms. Trimethoprim interferes with tetrahydrofolate synthesis by competing with dihydrofolate for binding to DHFR ( Fig. 3 ) and, consistent with our simple theory, is resisted by DHFR overexpression ( Fig. 2 , model i). Sulphonamides interfere with dihydropteroate (DHP) synthesis from pteridine diphosphate (PDP) and para-aminobenzoic acid (PABA) by competing with PABA for binding to the enzyme DHPS [43] , but are not resisted by DHPS overexpression ( Fig. 1b ). While trimethoprim renders DHFR catalytically inactive, sulphonamides, though considered ‘DHPS inhibitors’, do not inhibit catalysis by DHPS—instead, they are covalently attached to PDP in place of PABA [44] , [45] ( Fig. 3 ). The resulting dihydropterin–sulphonamide is not toxic to E. coli [45] , but this reaction wastes the essential metabolite PDP. We modelled PDP wasting by sulfamethoxazole by assuming that PDP is synthesized at a constant rate (by upstream components of the folate synthesis pathway) and consumed by DHPS to dihydropterin–sulphonamide or DHP. Strikingly, this model shows that when a drug induces a target-catalyzed reaction that wastes the target’s substrate, flux inhibition is independent of target concentration ( Fig. 2 , model w; Supplementary Methods ). The fraction of limiting substrate (for example, PDP) that is converted to the correct product (for example, DHP) is defined by the ratio of drug to drug-competing substrate (for example, sulphonamide to PABA ratio), weighted by binding affinity. This ratio is completely independent of the abundance of total enzyme or even uninhibited enzyme. This result is consistent with the observation that increased PABA synthesis confers sulphonamide resistance [46] and explains why, in contrast, increased expression of DHPS confers no such resistance. Further, this analysis reveals the previously unappreciated significance of the sulphonamide-PDP reaction: sulphonamides inhibit growth not by competitive inhibition of an essential enzyme, but by suicide inhibition of an essential metabolite, thereby wastefully diverting metabolic flux. 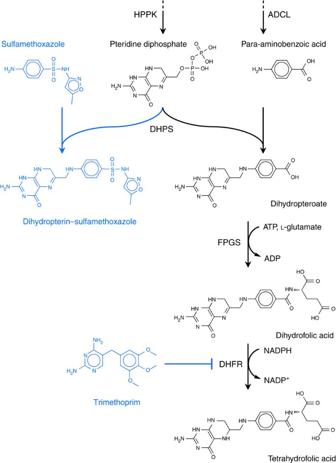Figure 3: Two different modes of folate synthesis inhibition demonstrate that target overexpression confers resistance to a drug that inhibits metabolic flux but not to a drug that diverts metabolic flux. Drug action on folate synthesis is shown in blue. Both trimethoprim and sulphonamides are considered ‘inhibitors’ of enzymes in the folate synthesis pathway, but while trimethoprim inhibits catalysis by competing with dihydrofolic acid for binding to Dihydrofolate reductase (DHFR), sulphonamides compete with para-aminobenzoic acid for binding to Dihydropteroate synthase (DHPS) and, rather than preventing catalysis, are covalently linked by DHPS to the substrate pteridine diphosphate. Our data and mathematical analysis show that this mechanistic distinction between flux inhibition or flux diversion leads to resistance by target overexpression for trimethoprim but not for sulphonamides. ADCL, aminodeoxy-chorismate lyase; FPGS, folylpolyglutamate synthetase; HPPK, 6-hydroxymethyl-7,8-dihydropterin pyrophosphokinase. Figure 3: Two different modes of folate synthesis inhibition demonstrate that target overexpression confers resistance to a drug that inhibits metabolic flux but not to a drug that diverts metabolic flux. Drug action on folate synthesis is shown in blue. Both trimethoprim and sulphonamides are considered ‘inhibitors’ of enzymes in the folate synthesis pathway, but while trimethoprim inhibits catalysis by competing with dihydrofolic acid for binding to Dihydrofolate reductase (DHFR), sulphonamides compete with para-aminobenzoic acid for binding to Dihydropteroate synthase (DHPS) and, rather than preventing catalysis, are covalently linked by DHPS to the substrate pteridine diphosphate. Our data and mathematical analysis show that this mechanistic distinction between flux inhibition or flux diversion leads to resistance by target overexpression for trimethoprim but not for sulphonamides. ADCL, aminodeoxy-chorismate lyase; FPGS, folylpolyglutamate synthetase; HPPK, 6-hydroxymethyl-7,8-dihydropterin pyrophosphokinase. Full size image Enhanced sensitivity to drugs that induce toxic reactions Having seen how two drugs that inhibit the same pathway can display different responses to overexpression of their targets, we next show how even two drugs with the same target can show opposite responses to target overexpression, reflecting differences in their mechanisms of action. Gyrase overexpression confers resistance to coumermycin A1 ( Fig. 1b ). However, overexpression of this same target actually confers sensitivity to ciprofloxacin (consistent with past predictions [47] and with observations in eukaryotic DNA topoisomerases [48] ). Coumermycin A1 competes with ATP binding and renders Gyrase inactive [36] , producing the behaviour predicted by the target-inhibition model ( Fig. 2 , model i). Conversely, ciprofloxacin only inhibits part of Gyrase’s function: ciprofloxacin contacts the DNA substrate and permits DNA cleavage by Gyrase but prevents re-ligation, thereby generating double-stranded DNA breaks [49] . Accordingly, growth inhibition by this class of drug (quinolones) correlates with the number of drug-stabilized DNA-Gyrase complexes [50] , and should therefore increase with Gyrase overexpression. We generalize this behaviour beyond DNA-damaging agents with a simple model of ‘toxic activity’, showing that when growth rate is any monotonic function of the number of drug-bound targets, IC50 depends inversely on fold overexpression of target ( Fig. 2 , model t; Supplementary Fig. 5 , Supplementary Methods ): Thus, when growth is inhibited by a toxic activity of a drug-bound target, rather than a lack of normal target activity, target overexpression enhances drug sensitivity instead of conferring resistance. Similar scenarios of toxic enzyme–drug complexes include the ‘translation-inhibiting’ aminoglycosides which when bound to the ribosome permit translation except with lethally severe mistranslation [51] , [52] , and pro-drugs that must bind an enzyme to be activated into a toxic form [53] . Consistent with the ‘toxic activity’ model, we observe an increase in sensitivity to the pro-drug nitrofurantoin with increasing expression of the drug-activating enzyme ( Supplementary Fig. 6 ). This study shows that increasing the expression of the drug’s target gene can have a wide range of effects on resistance to that drug; the simple expectation that resistance will monotonically increase is only one of several possibilities. However, these opposing complex responses of drug resistance to target overexpression can be fully rationalized by simple models with few assumptions that account for distinct molecular mechanisms of drug action and the possible fitness costs of gene overexpression ( Fig. 2 ). The contrasting effects of target overexpression on trimethoprim and sulfamethoxazole resistance, and on ciprofloxacin and coumermycin A1 resistance, illustrate a common principle: target overexpression may confer resistance to a drug that only inhibits target activity, but will not confer resistance to a drug that acts by inducing harmful target-catalyzed reactions. Importantly, even drugs that are ‘merely’ inhibitors at the molecular level may exert their cellular toxicity through harmful target-catalyzed reactions if they only partially inhibit target activity, as demonstrated by ciprofloxacin which inhibits Gyrase part of the way through its catalytic cycle. Such mechanisms might therefore be more widespread than is appreciated. The quantitative models employed here also clarify that the competitive or non-competitive nature of drug binding, previously hypothesized to define whether or not target overexpression confers resistance, is of no consequence ( Supplementary Methods , and consider sulphonamides as a counter-example). The general principles elucidated here should be applicable to growth-inhibitory drugs beyond antibiotics, including antimalarials, pesticides and cytotoxic chemotherapies, and may provide a conceptual framework also for dose-dependent gene–gene interactions. These results explain why only for some drugs can resistance evolve via target overexpression, and show that the common notion that drug resistance is positively related to target expression, upon which multiple approaches to target identification are based [14] , [17] , [18] , [19] , does not apply to important classes of drug mechanism. These mechanisms include, but may not be limited to, drugs that divert rather than inhibit metabolic flux and drugs that induce harmful target-catalyzed reactions. Another mechanistic distinction that can be made by target overexpression is that between an ‘inhibitor–target enzyme’ interaction and a ‘prodrug–activating enzyme’ interaction ( Supplementary Fig. 6 ). The potential for this distinction to go long undetected is exemplified by the recent discovery that the antitubercular agent para-aminosalicylic acid is a pro-drug activated by DHPS rather than a DHPS inhibitor [54] , [55] . The details of many drugs’ molecular mechanisms are unclear [56] and we may yet be surprised by misunderstood mechanisms. Thus target overexpression, while not always reliable for target identification, can provide a simple yet powerful approach to characterize a drug’s action on known or suspected targets, systematically distinguishing between simple inhibition and more complex molecular mechanisms. Strains and media E. coli strain BW25113 was the host for all studies. As lacZYA is deleted in BW25113, IPTG does not incur fitness costs for lacZYA production [30] , and graded induction is possible without the LacY permease, that would otherwise cause all-or-none induction of LacI-regulated promoters [57] , [58] . BW25113 was transformed with plasmid pCSλ, encoding a constitutively expressed bacterial bioluminescence operon [27] . Plasmids encoding each target gene (in a pCA24N backbone that also expresses lacI ) were obtained from the E. coli ASKA library (‘a complete set of E. coli K-12 Open Reading Frame archive’) [25] , a strain library where each full length open reading frame from E. coli W3110 is cloned into an expression vector. This study used the ASKA library without green fluorescent protein fusions. The selected ASKA plasmids were sequenced to confirm gene identity, and were transformed into BW25113 pCSλ. DNA Gyrase was expressed by encoding both subunits ( gyrA and gyrB ) on a single transcript—consisting of the 5′ untranslated region (UTR) and coding sequence of gyrA followed immediately by the 5′ UTR, coding sequence, and 3′ UTR of gyrB . This transcript was produced by PCR amplification (Phusion polymerase, New England Biolabs) of the desired regions of gyrA and gyrB from the chromosome of E. coli MG1655, isothermal assembly into the pCA24N plasmid backbone (Gibson Assembly Mastermix, New England Biolabs) and sequencing of the cloning junctions were done to confirm correct assembly. To accomplish this, the pCA24N backbone was amplified with primers 5′-CTGCAGCCAAGCTTAATTAGC-3′ and 5′-GAATCTATTATAATTGTTATCCGCTCAC-3′; gyrA was amplified with 5′-gctttgtgagcggataacaattataatagattcaattgCTTTGAATCCGGGATACAGTAG-3′ and 5′-ctcgctcatttatacttgggTTATTCTTCTTCTGGCTCGTCG-3′, where the lowercase letters are tags complementary to the ends of other PCR products in the isothermal assembly reaction; gyrB was amplified with 5′-cgacgagccagaagaagaaTAACCCAAGTATAAATGAGCGAG-3′ and 5′-agctcagctaattaagcttggctgcaggtcgacccTTAAATATCGATATTCGCCGCTTTC-3′. As carriage of this plasmid was found to lower growth rate even without IPTG induction, the high copy number colE1 origin of replication in pCA24N was replaced with the low copy number SC101 origin [59] , again via PCR amplification and isothermal assembly. For this reaction pCA24N- gyrAB was amplified with primers 5′-gcagcaaaacccgtaccctagAGCGCAGCGAGTCAGTGAG-3′ and 5′-cggattatcccgtgacaggtcatGATTATCAAAAAGGATCTTCACCTAGATCC-3′; and the pSC101 origin was amplified from pZS12 [59] with 5′-ggatctaggtgaagatcctttttgataatcATGACCTGTCACGGGATAATCCG-3′ and 5′-ctcactgactcgctgcgctCTAGGGTACGGGTTTTGCTGC-3′. Wildtype drug susceptibilities were determined using a matching strain with no additional drug target gene expression: BW25113 pCSλ pCA24N-Δpromoter- yfp for most drug targets, or BW25113 pCSλ pCA24N-SC101-Δpromoter- yfp for DNA Gyrase. In these plasmids, the IPTG-inducible promoter in pCA24N had been deleted, and yellow fluorescent protein was encoded in place of a drug target gene. All experiments were performed in M63 minimal medium (2 g l −1 (NH 4 ) 2 SO 4 , 13.6 g l −1 KH 2 PO 4 , 0.5 mg l −1 FeSO 4 7H 2 O, 1 mM MgSO 4 , adjusted to pH 7.0 with KOH) and supplemented with 0.2% glucose, 0.01% casamino acids, and 0.5 mg l −1 thiamine, and also 10mg l −1 chlorampenicol and 25 mg l −1 kanamycin for the maintenance of the pCA24N and pCSλ plasmids, respectively. Drug solutions were made from powder stocks (from Sigma Aldrich unless otherwise specified: cefsulodin, C8145; chloramphenicol, C0378; ciprofloxacin, 17850; coumermycin A1, C9270; IPTG, Omega Bio-Tek AC121; kanamycin, K1876; mecillinam, 33447; nitrofurantoin, N7878; ortho-nitrophenyl-β-galactoside, N1127; polymyxin-B, P0972; sulfamethoxazole, S7507; triclosan, TCI America T1872; trimethoprim, T7883). Drug and IPTG gradients were made by serial dilution in M63 medium. Growth rate assay The constitutive bioluminescence that results from pCSλ enables cell densities in growing cultures to be precisely measured over many orders of magnitude by photon counting [27] . Cultures were grown in black 96-well plates with white wells (Perkin Elmer 6005039) sealed with clear adhesive lids (Perkin Elmer 6005185). Wells contained 200 μl of media inoculated with ~100 to 300 cells from freshly thawed −80 ° C frozen cultures. Plates were grown in a 30 ° C room at 70% humidity, and growth was assayed by a Perkin Elmer TopCount NXT Microplate Scintillation and Luminescence Counter measured each well for 1 s. Experiments of 10–16 plates allowed each plate to be measured every 30–50 min. Plate stacks were ventilated by fans to eliminate spatial temperature gradients and ensure uniform growth conditions across each plate. In each experiment, distributed throughout the plate stack were three control plates of uniform media conditions to verify the absence of growth rate gradients within plates or across the plate stack. In Fig. 1b growth rates of wildtype under antibiotic treatment are the mean of 3–6 measurements, except DNA gyrase which is the mean of duplicates. Sixteen replicates of drug-free wildtype per assay plate provided confirmation that plate to plate variability in growth was <2%, permitting the ‘stitching’ together of multiple assay plates to measure growth versus expression over very wide ranges in drug concentration. Growth rate is the slope of the logarithm of photon counts per second (c.p.s. ), and is taken from the steepest line of best fit observed in any 6 h timespan; this time corresponds to five doublings of a healthy culture. The slope of the logarithm of c.p.s. is unaffected by changes in luminescence per cell, such as might result from antibiotic treatments or changes in gene expression [27] . Trend lines to experimental data in Figs 1b and 2c are B-splines (Wolfram Mathematica 8). Beta-galactosidase assay The transcription rates of genes encoded in the pCA24N plasmid at different IPTG concentrations were measured by kinetic beta-galactosidase (LacZ) assays of pCA24N- lacZ , using a method adapted from Dodd et al. [26] Liquid cultures of BW25113 pCA24N– lacZ were prepared in a 96-well plate in the same manner as for growth rate assays. The plate was incubated at 30 ° C with shaking until the plate average OD 600 equalled 0.1 (mid log phase), as measured by a Perkin Elmer Victor plate reader. To assay pCA24N-colE1- lacZ , 20 μl of each well was promptly transferred to the corresponding well of a microtiter plate pre-warmed to 30 ° C, in which each well contained 30 μl of sterile media and 190 μl of lysis/assay buffer, consisting of 100 mM Tris-HCl pH 8.0, 1 mM MgSO 4 , 10mM KCl, 1% v/v β-mercaptoethanol, 100 mg l −1 polymyxin-B and 850 mg l −1 ortho -nitrophenyl-β-galactoside. To assay pCA24N-SC101- lacZ , the procedure was identical except that instead of adding 20 μl of bacterial culture plus 30 μl of sterile media to the lysis/assay buffer, 50 μl of bacterial culture was added to better enable measurement of the lower LacZ activity of this lower copy number plasmid. The lysis/assay plate was transferred to a Tecan Sunrise plate reader in a 30 ° C room at 70% humidity, and OD 410 was measured every minute for 2 h, with 20 s of shaking between each reading. For each well, promoter activity in Miller Units was calculated from the slope of OD 410 versus time, multiplied by 200,000, divided by the OD 600 of the culture that was transferred to that well, and divided by the volume (in microlitre) of the culture assayed (20 μl for pCA24N-colE1- lacZ , 50 μl for pCA24N-SC101- lacZ ) ( Supplementary Fig. 1 ). Beta-galactosidase assays in the presence of partially inhibitory antibiotic doses ( Supplementary Fig. 2 ) were performed by the same procedures as above. The degree of growth inhibition in these experiments was determined by kinetic measurements of OD 600 in a Perkin Elmer Victor plate reader, to measure the relative growth rates of cultures with and without antibiotic. Similar to the drug-free assay, each set of cultures, in a given antibiotic dose and spanning a gradient of IPTG concentrations, was lysed and assayed when OD 600 reached 0.1. How to cite this article : Palmer, A. C. and Kishony, R. Opposing effects of target overexpression reveal drug mechanisms. Nat. Commun. 5:4296 doi: 10.1038/ncomms5296 (2014).